Catalytic enantioselective addition of Grignard reagents to aromatic silyl ketimines α-Chiral amines are of significant importance in medicinal chemistry, asymmetric synthesis and material science, but methods for their efficient synthesis are scarce. In particular, the synthesis of α-chiral amines with the challenging tetrasubstituted carbon stereocentre is a long-standing problem and catalytic asymmetric additions of organometallic reagents to ketimines that would give direct access to these molecules are underdeveloped. Here we report a highly enantioselective catalytic synthesis of N -sulfonyl protected α-chiral silyl amines via the addition of inexpensive, easy to handle and readily available Grignard reagents to silyl ketimines. The key to this success was our ability to suppress any unselective background addition reactions and side reduction pathway, through the identification of an inexpensive, chiral Cu-complex as the catalytically active structure. α-Chiral amines are ubiquitous building blocks in natural products, pharmacophores, agrochemicals and functional materials [1] . As a result, the production of these compounds is a prominent topic in organic chemistry, with broad industrial applications. One of the most straightforward and atom-efficient approaches for the synthesis of α-chiral amines is the catalytic enantioselective alkylation of imines [2] , [3] , [4] . Tremendous advances have been made in the catalytic asymmetric addition of carbon-based nucleophiles to imines derived from aldehydes (aldimines), affording α-chiral amines with trisubstituted carbon stereocentres [2] , [3] . However, the analogous alkylation reaction of ketimines, which leads to the formation of α-chiral amines with tetrasubstituted carbon stereocentres, has not been solved and remains a long-standing challenge [2] , [3] , [4] . The main factors responsible for the paucity of methods available for the asymmetric alkylation of ketimines are (i) their sterically more congested structures, (ii) the low reactivity of their C=N bonds (versus C=O in ketones and C=N in aldimines), and (iii) the fact that ketimines, unlike ketones exist as E or Z isomers. Altogether, these features render the enantiodiscrimination by the chiral catalyst and the reactivity towards the alkylation particularly difficult. Over the past decade, great effort has been put into the development of general protocols, but the main successes have been based on the use of stabilized nucleophiles, such as Strecker and Mannich-type reactions [2] , [3] , [4] . Methods involving non-stabilized nucleophiles remain significantly underdeveloped, with only a few reports to date. The main advances in this area have been achieved in the field of Rh- and Pd-catalysed addition of Csp 2 -nucleophiles to N -sulfonyl ketimines using boron reagents [5] , [6] , [7] . However, the addition of Csp 3 -nucleophiles is restricted to methylations and ethylations of a small set of ketimines using organozinc or organoaluminium reagents with Cu, Zr or Rh catalysts [8] , [9] , [10] . The highly reactive Grignard reagents are probably the most commonly used non-stabilized nucleophiles in both laboratory and industry [11] . Apart from being easy to handle, inexpensive and readily available, these organometallic reagents provide high atom economy due to the transfer of all alkyl groups when compared with organozinc or organoaluminium reagents. Furthermore, if used in the alkylation of ketimines, their high reactivity might be helpful to overcome the low reactivity of the latter. Despite these obvious advantages, and the plethora of methods employing Grignard reagents for catalytic asymmetric C–C bond formation with Michael acceptors [12] , [13] , [14] , aldehydes [15] and ketones [16] , [17] not a single catalytic asymmetric reaction involving the direct addition of Grignard reagents to ketimines has been reported. Thus, a general protocol for the catalytic enantioselective addition of Grignard reagents to ketimines would be an important step forward in the synthesis of α-chiral amines with tetrasubstituted carbon stereocentre. We decided to evaluate the use of Grignard reagents in the Cu-catalysed alkylation of ketimines derived from acylsilanes, in order to access chiral α-silyl amines with tetrasubstituted carbon stereocentre. Organic compounds with one or more carbon atoms replaced by silicon are increasingly popular in medicinal chemistry, because of several attractive characteristics of silicon atoms, such as their similar valency and tetrahedral bonding pattern, lipophilic nature and their low toxicity [18] . For instance, α-silyl amine motifs with trisubstituted carbon stereocentres were recently used in the synthesis of peptide isosteres and are also present in several effective proteolitic enzyme inhibitors [19] , [20] . In contrast, chiral α-silyl amines with tetrasubstituted carbon have not been investigated yet, due to a lack of synthetic methods to access them. So far, only a handful of examples of catalytic asymmetric synthesis of chiral α-silyl amines with trisubstituted carbon stereocentres have been reported [21] , [22] , [23] , [24] . For the formation of α-silyl amines with tetrasubstituted carbon stereocentre, no efficient methods have been developed yet, with two examples of racemic synthesis having been reported until now [25] , [26] . The only report [23] in which synthesis of chiral α-silyl amines with tetrasubstituted carbon was presented is based on silyl transfer strategy and describes few products with low yields (13–20%) and e.e.’s (60–79%). Here we report that Grignard reagents are suitable nucleophiles for highly enantioselective addition reactions to silylated ketimines, promoted by a copper-based chiral catalyst. This transformation allows to access wide variety of N -protected α-chiral silyl amines with tetrasubstituted carbon stereocentres. Optimization of the reaction conditions We set out by exploring the addition of n -hexylmagnesium bromide to N -tosyl silyl ketimines 1 , which were synthesized by condensation of para- toluenesulfonamide with the corresponding acylsilanes. 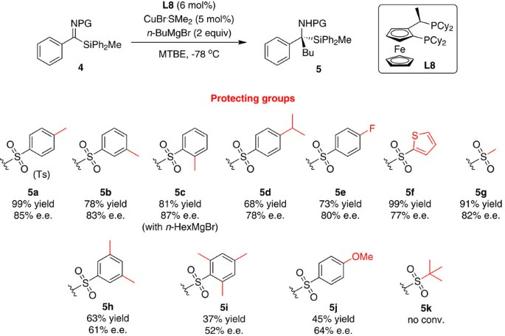Figure 1: Effect of the sulfonyl-protecting group. Evaluation of sulfonyl-protecting group on the reactivity of the ketimines and the enantioselectivity of the addition reaction. It is worth noting that all the ketimines prepared for this work were obtained with >95% E -configurational purity (see Supplementary Table 1 ). Aiming to overcome the low reactivity of the ketimine by use of highly reactive Grignard reagents, we also anticipated several potential problems in this system. The main complication in using Grignard reagents in addition reactions to ketimines is the control over the chemoselectivity: alkyl Grignard reagents with a hydrogen atom at the β-position bear the risk of reducing the ketimine substrate via β-hydride transfer, leading to the formation of undesired reduction side product, namely racemic secondary amine. This chemoselectivity issue can be further enhanced due to the bulkiness introduced by the silyl group, which might impede the formation of the hindered tetrasubstituted chiral carbon, and thus favour β-hydride transfer. To evaluate our reaction system we first treated N -tosyl silyl ketimine ( 1ab ) with n -hexylmagnesium bromide (2 equiv) in methyl tert -butyl ether (MTBE) at –78 °C ( Table 1 ). As expected, the blank reaction led mainly to the reduction product 3ab (addition:reduction=1:2) via β-hydride transfer (entry 1). To avoid the reduction pathway and at the same time activate the imine towards the addition of Grignard reagents, the optimization studies for the catalytic reaction were carried out in the presence of super-stoichiometric amounts of a mixture of BF 3 ·OEt 2 and CeCl 3 . This Lewis acid assisted synthesis was developed during our previous studies, where we found that a mixture of BF 3 ·OEt 2 and CeCl 3 prevents the undesired reduction pathway in the synthesis of tertiary alcohols [16] and that BF 3 ·OEt 2 can activate inherently unreactive substrates such as alkenyl-heteroarenes towards nucleophilic addition of Grignard reagents [14] . Table 1 Catalytic asymmetric alkylation of silyl ketimines: selected optimization results. Full size table The chiral catalytic systems screened in this study were comprises 5 mol% of CuBr·SMe 2 and 6 mol% of various chiral ligands. Using chiral ferrocenyl-based diphosphine ligand L1 the reaction proceeded fairly smoothly, with an addition to reduction ratio of 3:1 and a moderate 31% enantiomeric excess (entry 2). Preliminary optimization of the reaction parameters pointed to MTBE as a superior solvent to toluene, diethyl ether and dichloromethane (entries 2–5). Further ligand screening revealed biphenyl diphosphine-type ligand L2 and phosphoramidite-type ligand L3 to be inefficient (entries 6 and 7), while ferrocenyl ligand L4 outcompeted L1 both in reactivity and enantioselectivity and L5 in reactivity (entries 8 and 9). Next, we tested the steric effect of the silyl group on ketimines 1 . Substituting SiPhMe 2 ( 1ab ) for a bulkier SiPh 2 Me ( 1a ) group boosted the enantioselectivity drastically from 37 to 75% (entries 9 and 10). The ketimine with the smaller silyl group SiEt 3 ( 1ac ) afforded the product with an enantioselectivity comparable to that obtained with SiPhMe 2 (entry 11), while the ketimines 1ad and 1ae , with bulky SiPh 3 and SiPh 2 tBu groups were significantly less reactive (entries 12 and 13). Subsequently, a comprehensive ligand screening was carried out, customized to N -tosyl ketimine 1a , bearing a SiPh 2 Me moiety. Several ferrocenyl diphosphine ligands ( L5 – L8 ) led to product formation with satisfying yields and enantioselectivities (entries 14-17). The highest enantioselectivity (86%), as well as excellent reactivity and chemoselectivity, were obtained with the ferrocenyl ligand L8 (entry 17). We were delighted that an excellent addition to reduction ratio (22:1) could be obtained with this chiral ligand without the assistance of Lewis acids (entry 18). Effect of the sulfonyl-protecting group Following this, we shifted our focus to the effect of the steric and electronic properties of the nitrogen sulfonyl-protecting group on the reactivity of the ketimine and its enantioselectivity in the addition reaction ( Fig. 1 ). Various sulfonyl-protecting groups were evaluated in the addition of n -butylmagnesium bromide to ketimines 4 using the CuBr·SMe 2 / L8 catalytic system. Remarkably, our protocol tolerated a broad range of sulfonyl protecting groups. Aryl sulfonyl-protecting groups with a methyl substituent in para- , meta- or ortho- position of the aromatic group provided the corresponding products ( 5a, 5b and 5c , respectively) with comparable yields and enantioselectivities. Similarly, ketimines with the bulkier isopropyl or electron-withdrawing fluorine substituents in the para- position furnished the products 5d and 5e , respectively, with good yields and enantioselectivities. Both selectivity and reactivity were also found to be unabated when the aryl group was replaced by a thiophenyl or a methyl group (products 5f and 5g ). Increasing the bulkiness of the sulfonyl-protecting group by moving from 4-methyl to 3,5-dimetyl and 2,4,5-trimethyl substituted phenyl groups, led to a gradual decrease in both the reactivity of the ketimine and the enantiopurity of the products (compare 5a , 5h and 5i ). A relatively low yield and enantioselectivity were also obtained for the product 5j derived from the ketimine with the electron donating para -methoxy phenyl sulfonyl group. The introduction of a bulky tert- butyl sulfonyl-protecting group inhibited the reactivity of the ketimine completely ( Fig. 1 , product 5k ). Figure 1: Effect of the sulfonyl-protecting group. Evaluation of sulfonyl-protecting group on the reactivity of the ketimines and the enantioselectivity of the addition reaction. Full size image Ketimine substrate scope For the evaluation of the substrate scope we chose the reaction between N -tosyl silyl ketimines 1 and n -hexylmagnesium bromide ( n -HexMgBr) under optimized reaction conditions, namely 5 mol% of CuBr·SMe 2 , 6 mol% of L8 , 2 equiv of Grignard reagent, 1–10 h reaction time, –78 °C and MTBE as a solvent ( Table 2 ). The examination of a wide range of ketimines revealed that the reaction is remarkably general. With all examined ketimines we obtained mainly the desired addition product, providing the corresponding α-silyl amines with tetrasubstituted carbon stereocentre with excellent isolated yields, ranging from 77 to 99% and high enantioselectivities ranging from 70 to 94%. Table 2 Ketimine substrate scope. Full size table Halogen substituents (F, Cl, Br) in the meta - and para -positions of the aryl silyl ketimines were tolerated, and the corresponding products ( 6b, 6c, 6e–6h ) were obtained with high yields and enantiopurities (entries 2, 3 and 5–8). As expected, ortho -substituted aryl silyl ketimines were less reactive. Thus, the assistance of a Lewis acid mixture was required to obtain the corresponding ortho -F-substituted aryl silyl amine 6d in 87% yield and 70% e.e. (entry 4). In the case of para- and meta- trifluoromethyl substituted aryl silyl ketimines, the corresponding amine products 6i and 6j were obtained with high yields (89 and 77%) and e.e.’s (93% and 79%, entries 9 and 10). Ketimines with electron-donating para - and meta -methyl groups, as well as para - and meta -methoxy substituents, furnished the corresponding amines 6k–6n with good yields (72–83%) and enantioselectivities (82-87%) (entries 11–14). The reaction with another ketimine 1o , bearing a bulky, electron-donating tert- butyl group in the para -position afforded the corresponding alcohol 6o with a very good 87% yield and 91% e.e. (entry 15). In addition, high yields and enantioselectivities were obtained for amines 6p–6r derived from the corresponding para- and meta -OCF 3 and 2-naphtyl substituted ketimines 1p–1r (entries 16–18). Heteroaromatic substituent is also tolerated, as in the case of ketimine 1s , derived from 2-thiophenyl methyl ketone (entry 19). In order to access aliphatic amines, we attempted the synthesis of alkyl silyl ketimines, but were unable to obtain the corresponding substrates due to the low reactivity of the aliphatic acylsilane precursor. Thus, we decided to test instead aryl alkyl ketimine 1t , derived from 1-phenylbutan-1-one. A major issue of alkyl substrates, when used in combination with Grignard reagents, is the substrate enolization. Addition of HexMgBr to 1t using reaction conditions optimized for silyl ketimines furnished the desired product with low yield and nearly racemic. This is not surprising since the geometry of this substrate is very different from that of silyl ketimines. However, our preliminary optimization studies pointed that the enantioselective reaction with enolizable aryl alkyl ketimines is possible (90% yield and 65% e.e.) when a solvent mixture (MTBE/Et 2 O=1/1) and ligand L1 are used instead of the standard reaction conditions. All catalytic reaction were analysed after 10 h, to accommodate the reaction times required for the additions to ketimines with electron-donating groups. However, we noted that the reaction times for the additions to ketimines with electron-withdrawing groups were distinctly shorter (1 h to 4 h). Grignard reagent scope To complete the assessment of the scope of the reaction, we turned our attention to the Grignard reagents. A variety of Grignard reagents were examined under the optimized reaction conditions using meta -Cl substituted aryl silyl ketimine 1f as substrate ( Table 3 ). We were delighted to observe that our catalytic system, in contrast to previous reports on alkylations of ketimines [8] , [9] , [10] , was suitable not only for the addition of methyl and ethyl nucleophiles, but that longer alkyl chains were also tolerated. In general, we found that with an increase of the alkyl chain length, the enantioselectivity of the reaction increased as well. The addition of MeMgBr led to the corresponding amine 7a with excellent yield (92%) and 60% enantioselectivity (entry 1). Importantly, after a single crystallization, the enantiopurity of the amine 7a (found in mother liquor) was amplified to 96%, indicating a strong difference in solubility between the homo- and heterochiral species. Table 3 Grignard reagents scope. Full size table Increasing the chain length of the Grignard reagents to Et, n-Bu and n - Hex furnished the corresponding products ( 7b, 7c and 6f ) with high yields and enantioselectivities (entries 2–4). Product 7d , derived from the addition of δ-branched Grignard reagent was obtained with 97% yield and 90% e.e. (entry 5). The presence of an olefinic moiety or a chlorine atom in the Grignard reagents was also tolerated, demonstrating that functionalized amine products 7e – 7g can be obtained in high enantiopurity as well (entries 6–8). In our previous studies on the asymmetric addition of Grignard reagents to ketones, the more sterically hindered i -BuMgBr emerged as the optimal reagent in terms of yield and enantioselectivity [17] . Curiously, when we tested this reagent in the current reaction, no conversion of the ketimine substrate was observed, neither towards the addition or the reduction product. Similarly, no conversion was obtained with α-branched Grignard reagents (i-PrMgBr). We attribute this lack of reactivity towards bulky Grignard reagents to steric crowding of the silylated ketimine substrate. To examine the potential for the scaling up of these reactions, we performed a single experiment on a preparative scale (1 mmol) and were able to obtain the product 6e with excellent yield (90%) and enantioselectivity (91%), without any erosion from the original values obtained in the small-scale reaction ( Table 3 , entry 5). The cleavage of the N -tosyl protecting group, demonstrated with protected amine 6t , was achieved using Birch-type reduction. The free amine was obtained with 84% yield (product 8 , see Supplementary information / Supplementary methods ). Finally, we could also reduce the catalyst loading (to 1 mol% of CuBr·SMe 2 and 1.1 mol% of L8 ) and obtain 6f with only slight decrease of the yield (68%) and enantioselectivity (90%) compared with that obtained with catalyst loading of 5 mol% of CuBr·SMe 2 and 6 mol% of L8 ( Table 2 , entry 6). We have demonstrated that readily available and cost-efficient Grignard reagents are suitable nucleophiles for the highly enantioselective addition reaction to silyl ketimines, promoted by a copper-based chiral catalyst. This unprecedented transformation allows a highly efficient and enantioselective route to N -sulfonyl protected α-chiral silyl amines with tetrasubstituted carbon stereocentre. The feasibility of this approach for the synthesis of amines from enolizable aryl alkyl ketimines has been also demonstrated. This methodology offers an opportunity for future application of newly synthesized enantioenriched α-silyl amines in synthetic and medicinal chemistry. Furthermore, these results could herald a breakthrough in light of the broader paucity of methods for the catalytic enantioselective addition of Grignard reagents to ketimines. Application of the approach developed in this work to various kinds of ketimines is currently in progress. Copper-catalysed addition of Grignard reagents to silyl ketimines The general procedure is described for the synthesis of product 6e via the copper-catalysed alkylation of ketimine 1e with n -HexMgBr. A Schlenk tube equipped with septum and stirring bar was charged with ketimine 1e (0.1 mmol), CuBr·SMe 2 (0.005 mmol) and ligand ( S,R Fe )- L8 (0.006 mmol). Dry MTBE (2.5 ml) was added and the solution was stirred under nitrogen at room temperature for 10 min. Then the resulting solution was cooled to –78 °C and stirred for another 15 min. In a separate Schlenk tube, the corresponding Grignard reagent (0.2 mmol, 2M in Et 2 O) was diluted with MTBE (combined volume of 1 ml) under nitrogen and added dropwise to the reaction mixture during 40 min using a syringe pump. Once the addition was complete, the mixture was stirred for 10 h at –78 °C. The reaction was quenched with a saturated aqueous NH 4 Cl solution and the mixture was warmed to room temperature, diluted with dichloromethane and the phases were separated. The aqueous layer was extracted with dichloromethane (3 × 10 ml) and the combined organic layers were dried with anhydrous MgSO 4 , filtered and the solvent was evaporated in vacuo . Purification was performed by flash chromatography on silica gel using different mixtures of n -pentane:Et 2 O as the eluent and the enantiomeric excess was determined by chiral high-performance liquid chromatography analysis. Data availability The authors declare that the data supporting the findings of this study are available within the article and its Supplementary Information files. For the experimental procedures and spectroscopic and physical data of compounds, see Supplementary Methods . For NMR and high-performance liquid chromatography analysis of the compounds in this article, see Supplementary Figs 1–123 . The CCDC 1510318 ( 7a ) and CCDC 1510319 ( 1g ) contains the supplementary crystallographic data for this paper ( Supplementary Table 1 ). These data can be obtained free of charge from The Cambridge Crystallographic Data Centre via http://www.ccdc.cam.ac.uk/data_request/cif . How to cite this article : Rong, J. et al . Catalytic enantioselective addition of Grignard reagents to aromatic silyl ketimines. Nat. Commun. 7 , 13780 doi: 10.1038/ncomms13780 (2016). Publisher's note: Springer Nature remains neutral with regard to jurisdictional claims in published maps and institutional affiliations.